Secondary anionic phospholipid binding site and gating mechanism in Kir2.1 inward rectifier channels Inwardly rectifying potassium (Kir) channels regulate multiple tissues. All Kir channels require interaction of phosphatidyl-4,5-bisphosphate (PIP 2 ) at a crystallographically identified binding site, but an additional nonspecific secondary anionic phospholipid (PL(−)) is required to generate high PIP 2 sensitivity of Kir2 channel gating. The PL(−)-binding site and mechanism are yet to be elucidated. Here we report docking simulations that identify a putative PL(−)-binding site, adjacent to the PIP 2 -binding site, generated by two lysine residues from neighbouring subunits. When either lysine is mutated to cysteine (K64C and K219C), channel activity is significantly decreased in cells and in reconstituted liposomes. Directly tethering K64C to the membrane by modification with decyl-MTS generates high PIP 2 sensitivity in liposomes, even in the complete absence of PL(−)s. The results provide a coherent molecular mechanism whereby PL(−) interaction with a discrete binding site results in a conformational change that stabilizes the high-affinity PIP 2 activatory site. The eukaryotic inwardly rectifying potassium (Kir) channel family includes seven subfamilies expressed in tissues throughout the body and implicated in diverse physiological functions, such that mutations are causally linked to a number of metabolic and genetic diseases including diabetes, heart diseases, Andersen–Tawil syndrome and Epilepsy, ataxia, sensorineural deafness, tubulopathy syndrome [1] , [2] , [3] . Kir channels are regulated by diverse modulators including phosphorylation by protein kinase A, auxiliary proteins (sulphonylurea receptors, G protein βγ subunits), Na + , ATP, pore blockers (Mg 2+ , polyamine) [4] , [5] and ethanol [6] . However, and in common with many other channels and membrane proteins, all Kir channels require the binding of phosphatidyl-4,5-bisphosphate (PI(4,5)P 2 ; PIP 2 ) for activation [7] , [8] , [9] . The study of PIP 2 effects on ion channels has been facilitated by its low natural abundance (0.4~1.5% of anionic phospholipids) [10] and the availability of methods to manipulate PIP 2 concentrations in the membrane during electrophysiological experiments, either through enzymatic reactions or charge screening by specific antibodies or polycations [8] , [11] , [12] . Other anionic lipid species such as phosphatidylglycerol (PG), phosphatidic acid (PA), phosphatidylserine (PS), phosphatidylinositol (PI) and cardiolipin are also present at variable, and generally much higher, concentrations in native membranes [13] , [14] . Membrane lipid composition can vary under different physiological and pathological conditions [15] , [16] , [17] , and has been invoked causally in various diseases conditions [18] , [19] , [20] . However, progress in understanding the role of specific lipids in controlling of membrane protein function has been limited [21] because they cannot be readily manipulated in native membranes. Reconstitution of purified proteins in synthetic membranes makes it possible to study function in defined systems of known lipid and protein composition, and the availability of purified eukaryotic Kir2 channel protein, reconstituted into liposomes of defined composition has led us to the discovery that bulk anionic phospholipids are required in the membrane to generate the high PIP 2 sensitivity that is necessary for physiological activation [22] . Multiple anionic phospholipids (PL(−)s) including PG, PA, PS, PI and cardiolipin can fulfill this requirement, nonspecifically shifting PIP 2 sensitivity of Kir2.x channels by ~100-fold [22] . Increasing PL(−) in the membrane increases both channel open probability and unitary conductance [22] . Recent crystal structures of Kir2.2 and Kir3.2 channels reveal a defined PIP 2 -binding site and provide clues to how this binding may open the channel, but the nature of the PL(−)-binding site and the molecular mechanism of the synergistic effect on PIP 2 activation are unknown. Hansen et al. [23] showed that the anionic pyrophosphatidic acid (PPA) head group (−3 formal charge) can bind to essentially the same site as PIP 2 (refs 23 , 24 ). This observation might suggest that activatory PL(−)s bind to the same site as PIP 2 , although such a scenario provides no intuitive explanation for the synergistic effect of anionic lipids on PIP 2 action. Therefore, we began this study by characterizing the functional effect of PPA on Kir2.1 channel activation. We first showed that PPA is clearly inhibitory, with no detectable synergistic effect on PIP 2 activation. We then used extensive docking simulations of PL(−) head groups to identify a putative PL(−)-binding site that is formed by two lysine residues (K64 and K219) from two neighbouring subunits. The role of the two residues was examined experimentally through cysteine mutation and subsequent modification by an methanethiosulphonate (MTS) reagent containing a strongly hydrophobic moiety (a decyl chain). Neutralization of K64 and K219, by cysteine substitution reduces channel activity, but ‘lipid-tethering’ by modification of K64C with decyl-MTS strikingly induces high-affinity PIP 2 activation, even in the absence of PL(−). These functional assays implicate K64 as the primary residue for PL(−) interaction and pulling of the cytoplasmic Kir domain towards the membrane as the molecular mechanism underlying the PL(−) synergistic effect on PIP 2 -dependent channel activation. PPA is a competitive inhibitor of Kir2.1 channels Recently resolved crystallographic structures of chicken Kir2.2 (ref. 23 ) reveal a specific PIP 2 -binding site at the interface of the M2 helix and the cytoplasmic domain. These structures also show that an anionic lipid with a PPA head group (PPA) can bind at essentially the same site. This raises the possibility that the secondary requirement for anionic lipids to activate Kir2 channels [22] might be satisfied through binding to this site, perhaps if PIP 2 was only required at a subset of the subunits. Alternatively, PPA may act as either a competitive analogue or competitive antagonist of PIP 2 interaction and not as a secondary activator PL(−). To resolve these possibilities, the functional role of PPA was first determined. Purified wild-type (WT) Kir2.1 protein was reconstituted into liposomes of different lipid compositions. First, to test whether PPA could act as a PIP 2 analogue and activate channels in the absence of PIP 2 , liposomes were formed with PPA (zero, 0.1 or 1%), plus 10% 1-palmitoyl-2-oleoyl-sn-glycero-3-phosphoglycerol (POPG) (to supply the secondary nonspecific lipid requirement), and 1-palmitoyl-2-oleoyl-sn-glycero-3-phosphatidylethanolamine (POPE) for the remaining fraction of the lipid (here and in all further liposome experiments). As shown in Fig. 1a , PPA did not activate the channel under these conditions, suggesting that PPA cannot act as a functional substitute for PIP 2 . We then tested whether PPA could act as a PL(−) and suffice for the secondary anionic lipid effect in the presence of 0.1% PIP 2 . Although increasing POPG augmented channel activity as shown before [23] ( Fig. 1b ), PPA significantly decreased channel activity at all concentrations and channel activity was completely inhibited at >10% PPA. To further confirm the inhibitory effect of PPA, channel activity was measured in the presence of 0.1% PIP 2 , 10% POPG with or without additional 10% of either POPG or PPA ( Fig. 1c ). Although additional 10% POPG (that is, 20% total POPG) further enhanced activity ( P >0.05, one-way analysis of variance, Turkey’s honestly significant difference post hoc test), 10% PPA again completely abolished the channel activity. These results are reminiscent of competitive inhibition of PIP 2 -activated channel activity by other PIPs [22] , [25] and clearly show that PPA acts as a competitive inhibitor of PIP 2 and not as an activatory PL(−). 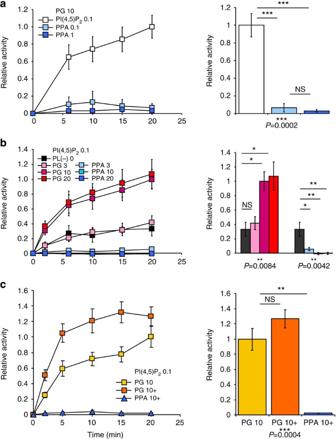Figure 1: PPA is a competitive inhibitor of PIP2(left)86Rb+uptake (normalized to maximum activity of WT Kir2.1 in 0.1% PIP2, 10% POPG). (Right) Maximum activity for 20 min. (a) Ten percent POPG was present in each case, and PPA or PIP(4,5)P2as indicated.n=3, mean±s.e.m.; ***,P<0.001 compared to the activity at PIP20.1 (P=0.0002, one-way analysis of variance (ANOVA), Tukey’s honestly significant difference (HSD)post hoctest). (b) PIP2(0.1%) was present in each case, and increasing POPG (pink) or PPA (blue) were added as indicated. Control experiment with no POPG or PPA is shown in black box.n=3, mean±s.e.m.; *,P<0.05 and **,P<0.001 compared to the activity at PL(−) 0 (P=0.0084 andP=0.0042, one-way ANOVA, Tukey’s HSDpost hoctest). (c) PIP2(0.1%) and 10% POPG were present in each case, with an additional 10% POPG (total 20%) or 10% PPA, as indicated.n=3, mean±s.e.m. **,P<0.01 compared to the activity at PG 10 (P=0.0004, one-way ANOVA, Tukey’s HSDpost hoctest). Figure 1: PPA is a competitive inhibitor of PIP 2 (left) 86 Rb + uptake (normalized to maximum activity of WT Kir2.1 in 0.1% PIP 2 , 10% POPG). (Right) Maximum activity for 20 min. ( a ) Ten percent POPG was present in each case, and PPA or PIP(4,5)P 2 as indicated. n =3, mean±s.e.m. ; ***, P <0.001 compared to the activity at PIP 2 0.1 ( P =0.0002, one-way analysis of variance (ANOVA), Tukey’s honestly significant difference (HSD) post hoc test). ( b ) PIP 2 (0.1%) was present in each case, and increasing POPG (pink) or PPA (blue) were added as indicated. Control experiment with no POPG or PPA is shown in black box. n =3, mean±s.e.m. ; *, P <0.05 and **, P <0.001 compared to the activity at PL(−) 0 ( P =0.0084 and P =0.0042, one-way ANOVA, Tukey’s HSD post hoc test). ( c ) PIP 2 (0.1%) and 10% POPG were present in each case, with an additional 10% POPG (total 20%) or 10% PPA, as indicated. n =3, mean±s.e.m. **, P <0.01 compared to the activity at PG 10 ( P =0.0004, one-way ANOVA, Tukey’s HSD post hoc test). Full size image Docking simulations identify a potential PL(−)-binding site We previously used docking simulations to identify the crystallographic PIP 2 -binding site (‘primary’ site) [23] as a main binding site for PIP 2 as well as an additional (‘secondary’) site, located at the interface between two adjacent subunits near the end of the slide helix and the apex of the βC-βD loop [26] . To determine potential docking sites for other anionic lipids, we have now performed extensive docking simulations of various lipids to Kir2.1, in both the absence (‘Apo-docking’) and presence (‘PIP 2 -bound-docking’) of PIP 2 at the crystallographic site. The searched space is shown in Fig. 2a,b ; the PIP 2 head group as located in the crystal structure (PDB 3SPI) was removed in the Apo-docking but present in PIP2-bound-docking below. Tested lipids included negatively charged PPA, PA, PG, PS as well as neutral phosphophatidylethanolamine (PE) and phosphatidylcholine (PC). Lipid head group structures and partial charges used for docking simulations are shown in Supplementary Fig. S1 . Accepted poses, based on appropriate orientation relative to the bilayer normal and proximity to the membrane (see Methods), were clustered using a K-clustering algorithm [27] . For each tested lipid, optimal clustering efficiency was achieved by division into two clusters (see Supplementary Fig. S2 and Methods), corresponding to the previously suggested primary and secondary phospholipid sites. As an illustrative example, every accepted (3,727 at primary and 758 at secondary out of 10,000) docked poses of PG is shown in Fig. 2c . 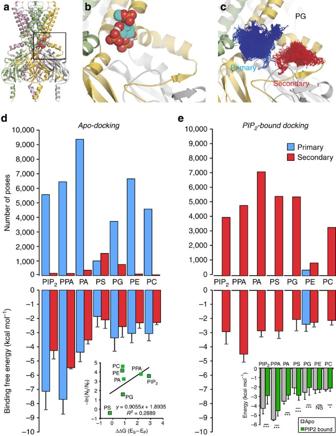Figure 2: Docking simulations of anionic lipids to Kir2.1 without or with PIP2pre-bound at the crystallographic site. (a) The tetrameric Kir2.1 homology model based on the PIP2-bound chicken Kir2.2 crystal structure (3SPI). Subunits are coloured in yellow, silver, pink and green in order. The PIP2ligand is shown in spheres at the crystallographic PIP2site. The space searched for docking simulations is marked by a black square, and in detail inb. (c) All accepted poses of PG in ‘Apo-docking’ are shown, subgrouped into two clusters: 3,727 poses are in the primary site (blue) and 758 poses in the secondary site (red). (d) Results from Apo-docking without crystallographic PIP2: the number and the mean binding free energy of accepted poses in primary (blue) or secondary (red) site are shown (mean±s.d.).ncorresponds to the number of accepted poses at each site shown in Table 1. Inset shows the energy difference between primary (EP) and secondary (ES) site versus inverse natural log of docking frequency ratio (NS/NP) between the two sites, which reasonably well follows the Boltzmann distribution. Data points refer to individual lipids from the Apo-docking simulation, and the line is the best fit to the data set. (e) Results (as ind) from PIP2-bound-docking simulated with PIP2pre-bound at the crystallographic-binding site (mean±s.d.). Inset shows the binding free energy at the secondary site from Apo- and PIP2-bound-docking, plotted for each lipid with their mean and s.d.ncorresponds to the number of accepted poses at the secondary site in the Apo- and PIP2-bound docking respectively shown in Table 1. The decrease in binding free energy is substantially significant (*,P<0.05 and ***,P<0.001 compared to the binding free energy in Apo-docking) for all anionic lipids determined by a two-tailed Student’st-test. Figure 2: Docking simulations of anionic lipids to Kir2.1 without or with PIP 2 pre-bound at the crystallographic site. ( a ) The tetrameric Kir2.1 homology model based on the PIP 2 -bound chicken Kir2.2 crystal structure (3SPI). Subunits are coloured in yellow, silver, pink and green in order. The PIP 2 ligand is shown in spheres at the crystallographic PIP 2 site. The space searched for docking simulations is marked by a black square, and in detail in b . ( c ) All accepted poses of PG in ‘Apo-docking’ are shown, subgrouped into two clusters: 3,727 poses are in the primary site (blue) and 758 poses in the secondary site (red). ( d ) Results from Apo-docking without crystallographic PIP 2 : the number and the mean binding free energy of accepted poses in primary (blue) or secondary (red) site are shown (mean±s.d.). n corresponds to the number of accepted poses at each site shown in Table 1. Inset shows the energy difference between primary (E P ) and secondary (E S ) site versus inverse natural log of docking frequency ratio ( N S / N P ) between the two sites, which reasonably well follows the Boltzmann distribution. Data points refer to individual lipids from the Apo-docking simulation, and the line is the best fit to the data set. ( e ) Results (as in d ) from PIP 2 -bound-docking simulated with PIP 2 pre-bound at the crystallographic-binding site (mean±s.d.). Inset shows the binding free energy at the secondary site from Apo- and PIP 2 -bound-docking, plotted for each lipid with their mean and s.d. n corresponds to the number of accepted poses at the secondary site in the Apo- and PIP 2 -bound docking respectively shown in Table 1. The decrease in binding free energy is substantially significant (*, P <0.05 and ***, P <0.001 compared to the binding free energy in Apo-docking) for all anionic lipids determined by a two-tailed Student’s t -test. Full size image In Apo-docking, all tested lipids, except PS, docked to the primary site with higher frequency and greater binding affinity compared with the secondary site ( Fig. 2d , top panel; Tables 1 and 2 ). The inconsistent behaviour of PS may originate from its unique zwitterionic head group structure with a positively charged amine and negatively charged carboxylic group. The relative distribution of docking events between the two sites was in reasonable agreement with the Boltzmann distribution, based on predicted binding free energies ( Fig. 2d , inset). Predicted binding at the primary site was much stronger for PIP 2 and PPA than for other lipids that at the primary site ( Fig. 2d ), but binding free energy at the secondary site was similar for all lipid species (maximum difference: 3.36 kcal mol −1 , mean±s.d. : −3.37±1.24 kcal mol −1 ), consistent with the relatively nonspecific and redundant character of the secondary PL(−)-activating effect [22] . Table 1 Number of accepted poses. Full size table Table 2 Binding free energy of accepted poses. Full size table We then carried out a series of docking simulations of the same lipids with PIP 2 pre-bound at the primary site (‘PIP 2 -bound-docking’; Fig. 2e ). In this situation, PIP 2 precluded additional binding of all but one of the lipids at the primary site and shifted binding almost exclusively to the secondary site, without substantially altering binding free energies at that site ( Fig. 2e ). PE was one exception in that it still docked to the primary site, essentially next to the PIP 2 head group, presumably facilitated by the small head group size and high charge density in the amine group. These simulations, using a rigid backbone model, therefore indicate that when PIP 2 is pre-docked at the primary site, the secondary site becomes the preferential site for PL(−) binding and no new sites become apparent. Two lysines are the main determinants of PL(−) interaction To identify residues that directly interact with lipids at the secondary site, hydrogen bonding between lipids and neighbouring residues was assessed ( Supplementary Table S1 ). 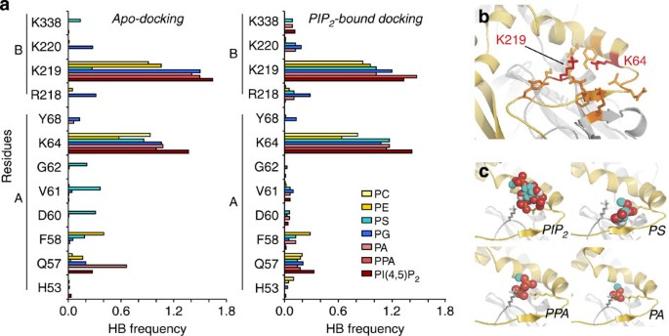Figure 3: Residue contributions to the secondary site. (a) Hydrogen bond frequency between all accepted poses and surrounding residues at the secondary site are shown for Apo- (left) and PIP2-bound-docking (right). All residues having H-bonding frequency >0.1 with any one of the tested lipids are shown. (b) Spatial location of the residues shown inaare depicted. The two residues, K64 and K219, of the highest contact frequency, are shown in red and others in orange. (c) Example structures of different lipids at the secondary site. K64, K219 and individual lipids (PIP2, PPA, PS and PA) are shown in stick and in atom colours. Figure 3a shows residues that have more than 10% hydrogen bond (H-bond) frequency out of all H-bonds detected between the accepted poses combined from Apo-docking (left) and PIP 2 -bound-docking (right) experiments. The H-bond frequency results were qualitatively similar for both cases, with two features of note. First, K64, at the N-terminal end of the slide helix of one subunit and K219 at the apex of the βC-βD loop of the adjacent subunit are the two key residues that make direct contacts with the docked lipids ( Fig. 3 ). In typical docked structures, these two positive side chains contributed to coordination of the negative phosphate group ( Fig. 3b,c ). Functional tests (below) demonstrate that these two residues are necessary for PL(−) activation and that chemical tethering of residue 64 to the membrane generates PL(−)-independent, high sensitivity to PIP 2 activation. Second, the residues found in the secondary site do not overlap with the residues forming the primary site ( Fig. 3b ). This observation demonstrates that the secondary site is indeed a unique and separate site from the primary PIP 2 -binding site. Figure 3: Residue contributions to the secondary site. ( a ) Hydrogen bond frequency between all accepted poses and surrounding residues at the secondary site are shown for Apo- (left) and PIP 2 -bound-docking (right). All residues having H-bonding frequency >0.1 with any one of the tested lipids are shown. ( b ) Spatial location of the residues shown in a are depicted. The two residues, K64 and K219, of the highest contact frequency, are shown in red and others in orange. ( c ) Example structures of different lipids at the secondary site. K64, K219 and individual lipids (PIP 2 , PPA, PS and PA) are shown in stick and in atom colours. Full size image Mutant channel activity is reduced in cell membranes To experimentally test the functional relevance of the secondary site as a nonspecific PL(−)-binding site, we mutated the K64 and K219 residues to cysteines, either individually (K64C, K219C) or together (K64/219C) in a ‘cysteine-less’ Kir2.1 background construct (CLS_Cont; see Methods). Both in vitro biochemical ( Supplementary Fig. S3 ) and mammalian cell-based ( Fig. 4 ) assays show that CLS_Cont is functionally equivalent to WT Kir2.1 channels. Mutant channel activity was first tested using a cellular 86 Rb + efflux assay ( Fig. 4a ) after transient expression in mammalian COSm6 cells ( Fig. 4a ). Although efflux rates were not different between WT Kir2.1 and CLS_Cont, each mutation substantially decreased channel activity, demonstrating that each residue is functionally important for maintenance of channel activity in mammalian cell membranes. 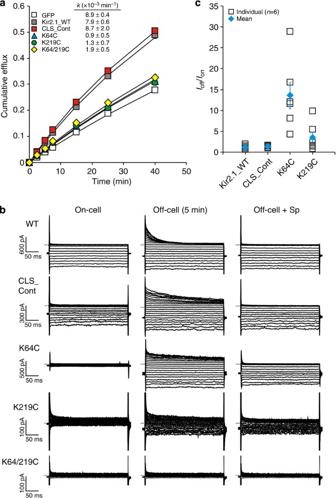Figure 4: Mutation of secondary site lysines inhibits channel activity in cell membranes. (a) Cumulative86Rb+efflux from Cosm6 cells versus time for WT (grey) and mutant Kir2.1 channels (CLS_Cont: red, K64C: blue, K219C: green, K64/219C: yellow). Nonspecific background flux was determined from GFP-transfected cells (white). Error bars are smaller than the symbols. Lines are the best fits of the single exponential equation described in the Methods, from which a rate constant (kin min−1) for each protein is obtained and shown in the figure. (b) Channel activity determined electrophysiologically on-cell (left), 5 min after excision (middle) and then in the presence of 10 μM spermine (right). (c) Current increase on patch excision (off-cell;Ioff) from cell-attached (on-cell;Ion) configuration. The fold-increase in current is shown for individual patches (white square), and mean and s.e. for each construct (n=6). Figure 4: Mutation of secondary site lysines inhibits channel activity in cell membranes. ( a ) Cumulative 86 Rb + efflux from Cosm6 cells versus time for WT (grey) and mutant Kir2.1 channels (CLS_Cont: red, K64C: blue, K219C: green, K64/219C: yellow). Nonspecific background flux was determined from GFP-transfected cells (white). Error bars are smaller than the symbols. Lines are the best fits of the single exponential equation described in the Methods, from which a rate constant ( k in min −1 ) for each protein is obtained and shown in the figure. ( b ) Channel activity determined electrophysiologically on-cell (left), 5 min after excision (middle) and then in the presence of 10 μM spermine (right). ( c ) Current increase on patch excision (off-cell; I off ) from cell-attached (on-cell; I on ) configuration. The fold-increase in current is shown for individual patches (white square), and mean and s.e. for each construct ( n =6). Full size image We carried out additional patch-clamp experiments on these transfected cells ( Fig. 4b ). In cell-attached patches, robust inwardly rectifying currents were measured through WT Kir2.1 as well as CLS_Cont channels. Following excision, channel currents were maintained, and typically increased slightly, as rectification gradually decreased because of slow loss of polyamines from within the recessed patch [28] . In contrast, inward rectifier currents were either very small, or undetectable, in cell-attached membrane patches in which mutant channel proteins (K64C, K219C and K64/219C) were expressed. Although K64/219C activity remained undetectable, spermine-sensitive inward rectifier currents slowly developed through K219C and especially K64C channels following patch excision, until current amplitudes were comparable to those measured from CLS_Cont patches ( Fig. 4b,c ). This remarkable behaviour demonstrates that channels are indeed present in the cell membranes but substantially closed when exposed to the intact intracellular milieu. The normal cytoplasmic environment is strongly reducing [29] , but membrane excision exposes the cytoplasmic face of the membrane to an oxidizing environment. Given the proximity of the two residues within the protein, K64C/K219C double mutants are likely to be disulphide bonded to each other (see Supplementary Fig. S4 ), but single mutant K64C and K219C will probably be reduced to free cysteines in the intact cell. They will be free to oxidize to surrounding proteins or lipids following patch excision, and we suggest that this oxidation then effectively tethers these residues to the membrane, thereby providing similar conformational energy to that which is normally provided by PL(−) interaction, to promote channel opening. This hypothesis is strongly supported by experiments below on recombinant channels in which the idea of ‘membrane tethering’ is directly assessed. Mutant channel activity is reduced in synthetic membranes Channel activities were also assessed from recombinant proteins incorporated into liposomes of defined lipid composition and in which nonspecific influence from cellular components is excluded. Control and mutant proteins were expressed in Saccharomyces cerevisiae , and then purified and reconstituted into liposomes with increasing POPG concentrations in the presence of constant 0.1% PIP 2 ( Fig. 5a , left). 86 Rb + influx into liposomes was measured as a function of time to assess channel activity. CLS_Cont protein showed essentially identical PL(−)-dependent activation ( Fig. 5a , left) to that of WT protein [22] ; activity reached maximum at ~10% POPG and there was no significant further activation at 20% POPG. Similar PL(−)-dependent activation was still observed but maximal channel activity was reduced slightly for the K219C mutant, markedly so for K64C, and there was no detectable activity from the K64C/K219C double mutant ( Fig. 5a , left). 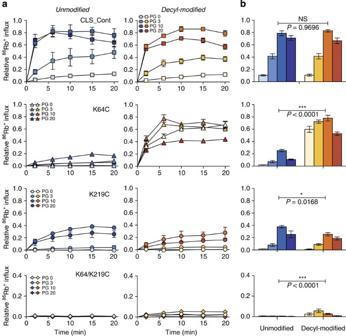Figure 5: Channel activation by decyl modification of secondary site residues. (a) Anionic lipid (PL(−))-dependent activation of CLS_Cont, K64C, K219C and K64/219C was determined without (left, blue colours) or with (right, red colours) modification by decyl-MTS by measurement of86Rb+uptake into liposomes. PIP2(0.1%) was present in all cases, and POPG varied as indicated.86Rb+uptake was normalized to the valinomycin count of the same sample. (b) Maximum channel activities with or without modification are plotted.n=6 (unmodified), 6 (modified) for CLS_Cont,n=6, 5 for K64C,n=6, 5 for K219C andn=6, 5 for K64/K219C. Error bars, s.e.m. *,P<0.05 and ***,P<0.001 compared to unmodified protein (two-way analysis of variance). Figure 5: Channel activation by decyl modification of secondary site residues. ( a ) Anionic lipid (PL(−))-dependent activation of CLS_Cont, K64C, K219C and K64/219C was determined without (left, blue colours) or with (right, red colours) modification by decyl-MTS by measurement of 86 Rb + uptake into liposomes. PIP 2 (0.1%) was present in all cases, and POPG varied as indicated. 86 Rb + uptake was normalized to the valinomycin count of the same sample. ( b ) Maximum channel activities with or without modification are plotted. n =6 (unmodified), 6 (modified) for CLS_Cont, n =6, 5 for K64C, n =6, 5 for K219C and n =6, 5 for K64/K219C. Error bars, s.e.m. *, P <0.05 and ***, P <0.001 compared to unmodified protein (two-way analysis of variance). Full size image Membrane tethering at secondary site restores channel activity Kir2 subfamily channels specifically require PI(4,5)P 2 for activation although all six other PIP species can interact with the PIP 2 site [22] , [26] , [30] , [31] . On the other hand, multiple different anionic phospholipids can satisfy the synergistic PL(−) effect with similar concentration dependence [22] . This suggests that the molecular mechanism exerted by PL(−) binding might be through a simple conformational change. We hypothesize this to be a generic pulling of the Kir domain towards the membrane. To directly test this idea, purified cysteine mutant and control proteins were modified in the detergent micelle state by decyl-MTS. This places a very hydrophobic 10-carbon acyl chain on modified cysteines, which will strongly partition into the membrane phase if appropriately located, as with modification of K64C and K219C. PL(−)-dependent activation of modified proteins was then again assessed using the 86 Rb + influx assay. Decyl modification did not affect CLS_Cont activation ( Fig. 5a , right), indicating that the expected disulphide bond (cystine) generated by the remaining two cysteines on the extracellular site of the protein remains as a disulphide bond. In contrast, decyl modification substantially increased the activity of single mutant K64C channels ( Fig. 5a , right) comparable to the activity of maximally active CLS_Cont channels (that is, in 0.1% PIP 2 plus 10% PG). Even more strikingly, marked channel activity was now present at zero POPG, R64C+decyl becoming almost PL(−) independent ( Fig. 5a , right). Decyl modification of K219C decreased maximum channel activity but had no significant effect on PL(−) dependence ( Fig. 5a , right). The double mutant (K64/K219C) was inactive before modification, but there was some low level of activity of decyl-MTS-modified channels ( Fig. 5a , right). We suggest that inactivity of the unmodified channels may be a result of disulphide bond formation between the two introduced cysteines. The low level of activity following decyl-MTS treatment was probably attributable to subsequent modification of a low level of reduced cysteines in the presence of dithiothreitol (<50 μM). Disulphide bond formation between the two introduced cysteines is supported by the presence of dithiothreitol-sensitive dimers of the double-mutant protein, but not CLS_Cont protein, in western blots ( Supplementary Fig. S4 ). Membrane tethering at secondary site enhances PIP 2 sensitivity In the absence of POPG or other PL(−), WT Kir2.1 channels are very weakly activated by supra-physiological levels of PIP 2 , whereas 25% PL(−) left-shifts PIP 2 sensitivity of human Kir2.1 channels by ~100-fold, making the channel fully active at only ~0.1% PIP 2 (ref. 22 ). If membrane tethering by decyl modification of K64C is functionally equivalent to the PL(−) interaction, then it should also cause left-shift in PIP 2 sensitivity of the modified channel in the absence of PL(−). To test this hypothesis, we assessed the POPG dependence of PIP 2 sensitivity in unmodified and decyl-modified K64C and K219C single mutants ( Fig. 6 ). The maximal activity of unmodified K64C and K219C mutants was lower than CLS_Cont but all showed a dramatic left-shift in PIP 2 sensitivity in the presence of POPG ( Fig. 6 , left). POPG dependence of PIP 2 sensitivity of CLS_Cont and K219C was unaffected by decyl-MTS treatment ( Fig. 6a–c , right). However, in striking agreement with the above prediction, the POPG-dependent shift was completely absent in decyl-modified K64C ( Fig. 6b , right), with the channels exhibiting identical high PIP 2 sensitivity in 0 or 10% POPG. This dramatic result not only suggests that K64 is the key residue for POPG interaction but also indicates that decyl modification of this residue can replace POPG interaction with this site to provide the membrane tethering that energetically sensitizes the channel to PIP 2 activation. 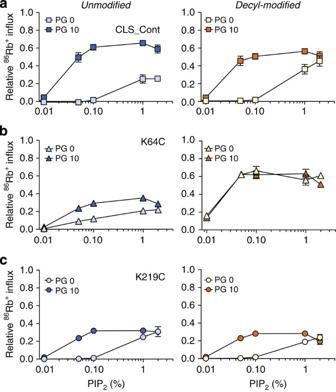Figure 6: Decyl modification abolishes PG-dependent shift of PIP2sensitivity activity-PIP2relationship for unmodified and decyl-modified CLS_Cont (a), K64C (b) and K219C (c) obtained from the maximum86Rb+uptake over the course of 20 min from experiments (as inFig. 5) with zero (light blue or yellow) or 10% (dark blue or orange) POPG. (n=3–6 in each case, mean±s.e.m.). Figure 6: Decyl modification abolishes PG-dependent shift of PIP 2 sensitivity activity-PIP 2 relationship for unmodified and decyl-modified CLS_Cont ( a ), K64C ( b ) and K219C ( c ) obtained from the maximum 86 Rb + uptake over the course of 20 min from experiments (as in Fig. 5 ) with zero (light blue or yellow) or 10% (dark blue or orange) POPG. ( n =3–6 in each case, mean±s.e.m.). Full size image It is becoming increasingly clear that the lipid components of the membrane are major regulators of the activity of ion channels [32] . Interaction with PIP 2 or related PIPs is essential for activation of many channels, including all Kir subfamily members [7] , [8] , [9] , and recent crystal structures have demonstrated a discrete binding site in Kir2.2 channels that underlies this effect, and provides significant insight to the molecular mechanism [23] . More generally mechanistic details of channel–lipid interactions are far from clear. The realization of obligate synergistic PL(−) regulation of PIP 2 -mediated Kir2.1 and Kir2.2 channel activation [22] indicates a previously unrecognized complexity, requiring the simultaneous binding of both lipids, a mechanistic scenario that is currently without explanation. Moreover, the relatively low affinity of PL(−) for this action suggests that, although the interaction is key for physiological channel activity, crystallographic resolution of the interaction may not be forthcoming. To gain further insight to the molecular basis of the PL(−) action, we therefore turned to the powerful approaches of molecular simulation, followed by experimental analysis using biochemical manipulation of channel structure. Using these approaches, we have successfully defined a discrete binding site for PL(−) that is both necessary and sufficient for PL(−) action, and a mechanism by which the interaction leads to PIP 2 sensitivity at physiological PIP 2 levels ( Fig. 7a ). 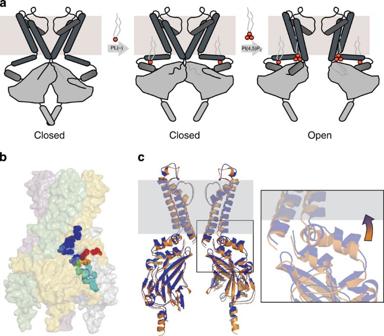Figure 7: Proposed model for secondary PL(−) regulation. (a) Hypothetical model: (i) in the absence of PL(−)s in the membrane, or when PL(−) interaction is lost by neutralization of the two positive charges at the secondary site, the cytoplasmic Kir domain is displaced from the membrane surface. (ii) The presence of PL(−)s in the membrane—or decyl modification of one of these—residues pulls the Kir domain closer to the membrane, which in turn induces conformational change in the primary site to generate high-affinity PIP2interaction. (iii) PIP2can then fully activate channels at low concentrations (0.05%). (b) The surface of Kir2.1 is shown with the same colour codes inFig. 2a. Residues (H53, R78, R80, K182, K185, K187 and K188) forming the primary site are shown in blue, and the secondary site (K64 and K219) in red. Residues implicated in interaction with other Kir channel modulators are also shown: L222 for cholesterol and Gβγ regulation are shown in green; the residues (F47, H42, L232, L245, P244, Y242, Y337 and L330) for ethanol and Gβγ are shown in cyan; N216 for Na+binding is shown in orange. (c) Structural models of Kir2.1 based on Kir2.2 bound to PIP2(3SPI, orange) and Kir3.2 additionally bound to Gβγ (4KFM, blue) to indicate potential motions associated with PL(−) interaction. Figure 7: Proposed model for secondary PL(−) regulation. ( a ) Hypothetical model: (i) in the absence of PL(−)s in the membrane, or when PL(−) interaction is lost by neutralization of the two positive charges at the secondary site, the cytoplasmic Kir domain is displaced from the membrane surface. (ii) The presence of PL(−)s in the membrane—or decyl modification of one of these—residues pulls the Kir domain closer to the membrane, which in turn induces conformational change in the primary site to generate high-affinity PIP 2 interaction. (iii) PIP 2 can then fully activate channels at low concentrations (0.05%). ( b ) The surface of Kir2.1 is shown with the same colour codes in Fig. 2a . Residues (H53, R78, R80, K182, K185, K187 and K188) forming the primary site are shown in blue, and the secondary site (K64 and K219) in red. Residues implicated in interaction with other Kir channel modulators are also shown: L222 for cholesterol and Gβγ regulation are shown in green; the residues (F47, H42, L232, L245, P244, Y242, Y337 and L330) for ethanol and Gβγ are shown in cyan; N216 for Na + binding is shown in orange. ( c ) Structural models of Kir2.1 based on Kir2.2 bound to PIP 2 (3SPI, orange) and Kir3.2 additionally bound to Gβγ (4KFM, blue) to indicate potential motions associated with PL(−) interaction. Full size image Our docking simulations identify two sites to which anionic lipids could bind ( Fig. 2 ). The first site (primary) at which the majority of docking events occurs corresponds to the PIP 2 site identified in X-ray crystal structures [23] , [24] . This agreement supports our Kir2.1 homology model and the parameters for ligand and docking simulations. When both this and an additional distinct PL(−)-binding (secondary) site are available, almost all lipids dock preferentially to the primary site ( Fig. 2d ), but if the primary site is occupied by PIP 2 , the secondary site becomes the most frequently docked site ( Fig. 2e ). Conversely, if the secondary site is pre-occupied by PIP 2 , 100% of PIP 2 docking is to the primary site, indicating that the secondary site is a spatially separate site to which anionic lipids can bind, such that even two PIP 2 molecules can bind to the two sites simultaneously ( Fig. 2e ). Two important experimental features of the synergistic PL(−) effect [22] further support this argument. First, the calculated binding free energies at the secondary site vary little between test lipids (maximum difference: 3.37 kcal mol −1 , mean±s.d. : −3.21±1.24 kcal mol −1 ), much less than the variability of binding free energies at the primary site (maximum difference: 5.84 kcal mol −1 , mean±s.d. : −4.37±2.22 kcal mol −1 ; Table 2), consistent with the experimental finding that the secondary PL(−) effect is nonspecific and that the efficacy of different lipids are similar [22] . Second, high-affinity PIP 2 sensitivity is specific, no other phospholipids can substitute. In Apo-docking experiments the binding affinity of PIP 2 and of the competitive antagonist PPA were both much higher at the primary site than that of other anionic phospholipids ( Fig. 2d ). Interestingly, the pre-occupancy of PIP 2 at the primary site actually increases the efficacy of PL(−) binding at the secondary site. PIP 2 at the primary site may create a negative electric potential that prevents the binding of negative lipid to other locations of weaker binding free energy, thereby restricting binding to the secondary site, that is, the next available high-affinity site. It also seems likely that the strong negative charges of PIP 2 and PPA are most sensitive to the negative electric potential generated by PIP 2 at the primary site; the binding free energy of most lipids at the secondary site was diminished but the reduction was greatest for PIP 2 and PPA, which brought the binding free energies of all tested lipids at the secondary site to within 3.37 kcal mol −1 of each other ( Fig. 2e , inset). This may explain why PIP 2 is not more efficient than other PL(−) at this action; 10% PIP 2 is required to activate channels as much in zero POPG [22] , as 10% POPG activates channels in 0.1% PIP 2 (ref. 22 ) ( Fig. 6a ). Similar binding energies for both lipids at the secondary site provide a simple interpretation of their nonspecific and similar efficacy. The secondary PL(−)-binding site overlaps with likely sites for allosteric regulation by Na + (refs 24 , 33 ), cholesterol [34] , [35] and Gβγ [8] that have been identified in other Kir channels. Na + increases the PIP 2 sensitivity of Kir3.2 and Kir3.4 channels, binding in an analogous pocket generated by carbonyl oxygen atoms of the βC-βD loop and the D226 side chain (see Fig. 7b ). The side chain of L222 in Kir2.1 (shown in green in Fig. 7b ), located at the βC-βD loop, points towards the interior of the large β sheet of the Kir domain and is spatially close to where Na + binds in Kir3.2. Although cholesterol inhibits WT Kir2.1 channels [34] , [36] , mutation of this particular residue (L222I) abolishes cholesterol sensitivity [35] , and mutation of the equivalent residue (I229) of Kir3.4 to leucine results in constitutively active channels in the absence of Gβγ (ref. 8 ). Other residues in the βC-βD loop are recognized to be involved in ligand regulation of other subfamily members. The same region (cyan Fig. 7b ) is implicated in a common binding site for alcohol [6] , as well as Gβγ (ref. 37 ) and Gα i/o (ref. 38 ) for allosteric regulation of Kir3 channels. Convergence of allosteric sites is very consistent with the idea that they all regulate sensitization to PIP 2 activation. The proposed secondary site was experimentally tested through single or double mutation of the two lysine residues. In intact cells, both single and double mutations of K64 and K219 significantly decreased channel activity, although channels are evidently in the membrane and can spontaneously activate following patch excision ( Fig. 4 ). In purified proteins, the effect of the individual mutations is predominantly to reduce lipid sensitivity, in a manner consistent with loss of PL(−) binding and loss of allosteric stabilization of the PIP 2 interaction. Modification with decyl-MTS, which covalently attaches a 10-carbon acyl chain to the cysteine sulfhydryl group, dramatically enhances channel activity of the K64C mutant and effectively maximally enhances PIP 2 sensitivity even in the complete absence of PL(−), thus indicating that decyl modification of K64C is functionally equivalent to PL(−) interaction ( Fig. 5 ). These equivalent effects of decyl-MTS modification and PL(−) interaction at the secondary site on PIP 2 sensitivity support the hypothesis that PL(−) interactions nonspecifically act to tether the cytoplasmic Kir domain, specifically the N-terminal slide helix, to the membrane and that it is this conformational effect that serves to increase PIP 2 affinity and stabilize the open state, as other allosteric regulators do [39] , [40] ( Fig. 7a ). Vertical motion or tethering of the cytoplasmic domain to the membrane seems to be a critical step for Kir channel opening [40] , [41] , [42] . Direct support for this idea comes from Kir2.2 crystal structures generated either in the absence [43] or presence [23] of anionic lipids (PIP 2 and PPA). These show marked differences in the location of the Kir domain relative to the potential membrane surface. In PIP 2 -bound structures, the C-linker adopts an α-helical conformation and the Kir domain is pulled towards the potential membrane surface by ~6 Å, relative to the Apo structure [23] . Comparison of recent Kir2.2 and Kir3.2 channel structures show that the additional binding of the allosteric regulator Gβγ to Kir3.2 further pulls the slide helix towards the membrane (4KFM) [44] relative to the PIP 2 -bound Kir2.2 structure (3SPI) [23] . Figure 7 C shows Kir2.1 homology models based on these two structures to illustrate potential motions coupled to PL(−) interaction. Rotation of the cytoplasmic domain with respect to the membrane as a result of Gβγ binding is suggested to be part of the gating mechanism [44] , [45] and may well occur with PL(−) binding to Kir2 channels, although our experiments cannot address this possibility. Pulling of the Kir domain of bacterial Kir channels (KirBac1.1) through membrane tethering also affects channel activity [46] . In this case, membrane tethering by decyl-MTS modification of introduced cysteines in the N-terminus or C-terminus ends of the slide helix resulted in opposite effects on KirBac1.1 activity, with tethering of the N terminus (R49C, that is, away from the pore axis) augmenting the channel activity, and tethering of the C terminus (L56C, close to the pore axis) reducing channel activity [46] . It is noteworthy that R49 of KirBac1.1 is structurally quite close to K64 of human Kir2.1, although these residues do not align exactly ( Supplementary Fig. S5 ). Moreover, recent analysis of sequence elements affecting PL(−) activation of KcsA indicates residues in exactly the same N-terminal slide helix region [47] . These results suggest that cytoplasmic domain tethering to the membrane through PL(−) binding at the secondary site may be a broadly conserved gating mechanism shared between pro- and eukaryotic K + channels. The K64 and K219 residues are loosely conserved among the seven eukaryotic Kir channel subfamilies ( Supplementary Fig. S5 ). Kir2 and Kir4 channels contain both lysines, Kir1 and Kir6, and Kir7 subfamily members have one or other of the two basic residues and Kir3 and Kir5 channels contain neither. Interestingly, physiologically, Kir5 subunits only appear to form functional channels as heterotetramers with Kir4 subunits [48] , and PL(−) regulation might then be conferred on the channels by the Kir4 subunits. As discussed above, Kir3 channels exhibit allosteric regulation of PIP 2 activation by other modulators, including Gβγ and Na + . It seems possible that these other modulators may convey the same effect on GIRK channels that PL(−) has on Kir2 channels, consistent with the cytoplasmic domain, and in particular the N-terminal slide helix, being pulled towards the membrane in the Gβγ-bound crystal structure [44] ( c.f. Fig. 7c ). Human Kir2.1 protein purification WT and mutant Kir2.1 proteins, tagged by Flag-His8 peptide at the C terminus, were expressed in and purified from the FGY217 strain of S. cerevisiae [49] . Expression levels and purification yields were similar for WT and mutant proteins. Mutagenesis was performed using QuickChange II site-directed mutagenesis kits (Stratagene Cloning Systems, CA) and verified by sequencing. Cysteine-less mutant Kir2.1 (CLS_Cont) was generated by introduction of a series of mutations: C43S, C54V, C76V, C89I, C101L, C149F, C169V, C209S, C311A, C356S and C375S. The two remaining cysteines (C122 and C154) are known to form a very stable intrasubunit disulphide bond [50] and were not substituted to maintain functional channels. 86 Rb + uptake assay Channel activity was assessed by 86 Rb + uptake into proteoliposomes [25] . POPE and POPG lipids were dissolved at 10 mg ml −1 concentration in buffer A (450 mM KCl, 10 mM HEPES, 4 mM NMG, pH 7.4) with 35 mM CHAPS. PIP 2 was solubilized at 1 mg ml −1 concentration in 10 mg ml −1 POPE solution. One milligram of lipid mixture in 100 μl was incubated at room temperature for 2 h, and 5 μg of protein was added and incubated for another 20 min. A lipid–protein mixture was run through partly dehydrated G-50 beads pre-equilibrated by buffer A containing additional 0.5 mM EGTA, which led to proteoliposome formation. Then, the proteoliposomes were run through partly dehydrated G-50 beads pre-equilibrated by buffer B (400 mM sorbitol, 10 mM HEPES, 4 mM N -methyl- D -glucamine, 0.5 mM EGTA, pH 7.4) to remove external KCl. Four hundred microlitres of buffer C containing 86 Rb + (PerkinElmer, Waltham, MA) at ~4.5 nCi was added at time zero. Equal amount of sample (60 μl) was collected and run through cation exchange beads where the trace amount of 86 Rb + in the external solution was captured by the beads. Uptake was measured over the first 20 min after commencing the assay and normalized to the maximum uptake in valinomycin. In Fig. 1 , the relative channel activity was obtained by renormalizing to the maximum activity of WT Kir2.1 in optimal lipid composition of 0.1% PI(4,5)P 2 , 90% POPE and 10% POPG. For cysteine modification, 100 μM Decyl-MTS (Toronto Research Chemicals, Ontario, Canada) was added to protein–lipid mixtures and incubated for 15 min before proteoliposomes were formed by passage over a size-exclusion column [46] . Brain PI(4,5)P 2 , POPE, POPG, dioleoylglycerol pyrophosphate (PPA) were purchased from Avanti Polar Lipids. 86 Rb + efflux assay COSm6 cells in 12-well plates were transfected with plasmids (400 ng) carrying Kir2.1 constructs cloned into pcDNA3.1(−), and pGreenLantern green fluorescent protein (GFP; 100 ng; Life Technologies, Grand Island, NY) mixed with Fugene 6 (Promega, Madison, WI) and cultured for an additional 24 h. New culture medium containing 1 μCi ml −1 86 RbCl was added, cells were incubated for a further 12 h and then washed twice with Ringer’s solution composed of (in mM) 118 NaCl, 2.5 CaCl 2 , 1.2 KH 2 PO 4 , 4.7 KCl, 25 NaHCO 3 , 1.2 MgSO 4 and 10 HEPES (pH 7.4). Ringer’s solution was repeatedly added and removed to collect released 86 Rb + from cells at 2.5, 5.0, 7.5, 15, 25 and 40 min time points ( t ). Finally, cells were lysed by 2% SDS solution to collect the remaining 86 Rb + within the cells. Cumulative efflux ( J ) relative to total 86 Rb + counts was computed to determine macroscopic channel activity. The channel-specific rate constant ( k 2 ) of transfected channel proteins was determined by fitting the data using MATLAB (Mathworks, Natick, MA) with the following equation, as described before [51] , , where rate constant k 1 , obtained from cells transfected with GFP alone, reflects endogenous background channel activity, and t is time. Electrophysiology COSm6 cells between passages 10 and 30 were grown on glass cover slips in 40-mm six-well plates and transiently transfected after reaching ~30–50% confluency. Each well of cells was transfected with 200 ng of GFP and 800 ng of the corresponding Kir2.1 plasmid using Fugene6 and used for electrophysiological experiments 24–48 h thereafter. Current responses were recorded with electrodes pulled from plain glass capillaries with a resistance of 1–4 MΩ and were filled with a buffer (K int ) containing (in mM) 140 KCl, 1 EGTA, 1 K 2 -EDTA, 4 K 2 HPO 4 and adjusted to pH 7.3 (KOH). Symmetrical K int solutions, also containing 10 μM spermine (Fluka, St. Louis, MO), were applied with a lightly pressurized perfusion system. Current responses were first elicited in the cell-attached patch-clamp configuration with a holding potential of −50 mV and pulsed for 300 ms to voltages between −100 and +100 mV at 10 mV increments. The patch was then excised to the inside-out patch-clamp configuration and moved between various solutions; the voltage step protocol was performed at regular intervals. Currents were low-pass filtered at 1 kHz (Axopatch 1D), sampled at 10 kHz (Digidata, 1200) and converted to digital files in Clampex7 (Molecular Devices) and stored on an external hard drive for offline analysis using Clampfit 10.3 (Molecular Devices). Homology modelling of human Kir2.1 channels Homology models of human Kir2.1 were built based on the chicken Kir2.2 (PDB 3SPI) crystal structure [23] . Human Kir2.1 is 76% and ~90% conserved relative to chicken Kir2.2. Sequence alignment was performed using the ClustalW webserver [52] and is shown in Supplementary Fig. S5 . One hundred homology models were generated through random seeding using the MODELLER 9.10 program [53] . Because of high sequence homology, modelled structures had identical backbone structures but with various rotamer orientations. PDBQT structure files, containing charge and atom type information, were generated from the PDB file of every homology model beginning with protonation, assigning Gasteiger charge [54] , merging of nonpolar hydrogen to the bonded carbon atom, and assigning atom type using Autodock Tool (ADT) 1.5.4 (ref. 55 ), and then the protein was aligned to the initial crystal structure using MacPyMOL programs (Schrödinger, New York, NY) to ensure that the docking search area was consistent among models. Docking simulations The head groups are critical determinants for lipid interactions with the Kir protein, and to facilitate simulations, essentially only the head group was modelled, including up to the first carbon atom of the glycerol moiety. Atom charges for PI(4,5)P 2 were obtained as published [56] and the charges for other anionic lipids were taken from the CHARMM force field [57] shown in Supplementary Fig. S1 . The atom charge of pyrophospatidic acid (PPA) was kindly provided by Wonpil Im (University of Kansas). ADT 1.5.4 was used to assign the atom type and torsion tree of each ligand [55] . The searched region fully covered the slide helix, the lower end of the TM1 helix, the N-terminal β-strand of subunit B (yellow) and the adjacent part of neighbouring subunits A (green) and C (silver), which was necessary for identification of potential interactions at the subunit interface as shown in Fig. 2b . The parameters for the grid map generation and docking simulations were the same as used previously [26] using AutoDock-4.2.3 (ref. 58 ). Each docking simulation was run for ~8 h on a single processor of the local IBM x3650-m 2 . For each template, 10,000 poses were generated for each ligand. Poses were accepted based on their orientation and relative location with respect to the potential membrane. First, a pose was accepted if the angle between the molecular vector that is designated for each lipid ( Supplementary Fig. S1 ) and the bilayer normal was less than 90°, that is, as will occur when the head group is either pointing away from the membrane or less than parallel to the membrane surface. Structural analysis was performed using in-house codes for MATLAB. The potential membrane surface was approximated by the centre of the slide helix based on studies of the binding of melittin (an amphipathic α-helix) to membranes [59] , [60] . If the primary phosphate that is directly connected to the lipid tails was located deeper than 4.5 Å into the membrane, or more than 8 Å from the surface of the membrane (defined by the centre of the slide helix), the pose was rejected. To elucidate representative binding sites, accepted poses were clustered into subgroups. A K-mean clustering algorithm [27] was adopted using the root mean squared deviation of the phosphorus atom position as a metric. The number of clusters for each ligand was determined to minimize the performance index ( Q ) [61] . The smaller the Q value, the greater the inter-subgroup variance and the smaller the intra-subgroup variance, which indicates better clustering performance (see Supplementary Fig. S2 and text). To determine the residues involved in ligand binding, hydrogen bonds were postulated based on the two following criteria [62] : first, the distance between the donor and acceptor atoms being shorter than or equal to 3.4 Å and second, the angular orientation being smaller than or equal to 30° between the two unit vectors. One joins hydrogen bond donor atom and hydrogen atom and the other joins hydrogen bond donor and acceptor atoms. Contact frequency was determined by counting the number of observed hydrogen bonds and dividing this by the total number of poses in each cluster. Statistical analysis Statistical significance was analysed using an unpaired t -test and either one-way or two-way analysis of variance as appropriate. Statistical significance of P <0.05, P <0.01 and P <0.001 is indicated by single, double and triple asterisks, respectively. How to cite this article: Lee, S.-J. et al. Secondary anionic phospholipid binding site and gating mechanism in Kir2.1 inward rectifier channels. Nat. Commun. 4:2786 doi: 10.1038/ncomms3786 (2013).